Dissecting the role of aberrant DNA methylation in human leukaemia Chronic myeloid leukaemia (CML) is a myeloproliferative disorder characterized by the genetic translocation t(9;22)(q34;q11.2) encoding for the BCR-ABL fusion oncogene. However, many molecular mechanisms of the disease progression still remain poorly understood. A growing body of evidence suggests that the epigenetic abnormalities are involved in tyrosine kinase resistance in CML, leading to leukaemic clone escape and disease propagation. Here we show that, by applying cellular reprogramming to primary CML cells, aberrant DNA methylation contributes to the disease evolution. Importantly, using a BCR-ABL inducible murine model, we demonstrate that a single oncogenic lesion triggers DNA methylation changes, which in turn act as a precipitating event in leukaemia progression. Genetic alterations impairing cellular differentiation and growth control are widely regarded as the molecular causes of chronic myeloid leukaemia (CML) and acute myeloid leukaemia [1] , [2] , [3] . Recent evidences suggest that epigenetic alterations such as DNA methylation can contribute to leukaemia pathogenesis [4] , [5] , [6] . In particular, abnormal epigenetic regulation of specific genes might play an important role in both leukaemia development and therapeutic responsiveness. CML is a particular type of leukaemia characterized by the presence of the BCR-ABL oncogene. BCR-ABL is a constitutive active tyrosine kinase mediating the deregulation of several pathways involved in proliferation and differentiation [7] . Although the expression of BCR-ABL is considered the primarily feature associated with CML onset, other molecular mechanisms contributing to CML development remain to be elucidated. Both hypermethylation of specific genomic loci and genome-wide hypomethylation have been found to correlate with cancer development. Specifically, hypermethylation of tumour suppressor genes has been found to play a crucial role in carcinogenesis by affecting normal cell growth [8] . Further, aberrant DNA methylation has been linked to the onset of leukaemic clones resistant to tyrosine kinase inhibitors and deemed responsible for CML propagation and progression [9] . Among the genes found to be hypermethylated in CML and other lymphoid malignancies, and correlating with a poor outcome, are HOXA4 and HOXA5 , both acting as differentiating genes during hematopoiesis [10] . Interestingly, the observation that a member of CCAAT/enhancer-binding protein ( CEBP ) family of transcription factors: DNA damage-inducible transcript 3 (DDIT3 gene, hypermethylated in CML [11] , suggests that the aberrant epigenetic regulation of the CEBP ) gene may also play a role in leukaemia onset [12] . Taken together, these findings indicate that aberrant DNA methylation might contribute to leukaemia development by synergizing with acquired genetic lesions. However, the lack of suitable animal models or other tools to directly address this particular question has constrained a thorough analysis. Human-induced pluripotent stem (iPS) cells can be generated from various cell types, including cancer cells, by overexpressing a defined set of transcription factors including OCT4, SOX2, KLF4 and c-MYC (refs 13 , 14 , 15 , 16 , 17 ). Previous studies have shown that cellular reprogramming might be able to erase tissue-specific DNA methylation and to re-establish an embryonic stem (ES)-like DNA methylation state [18] . Here by means of cellular reprogramming followed by in vitro re-differentiation we tested the functional relevance of DNA aberrant methylome in CML development. Reprogramming of CML cells into an iPS-like state was able to erase the cancer-specific DNA methylation signature and to identify a cell population no longer effective in producing CML when subsequently transplanted into immunocompromised mice. Finally, using an inducible BCR-ABL transgenic mouse [19] , we demonstrate in vivo that a single genetic aberration perturbing DNA methylation profile acts as a crucial precipitating event in CML disease development. Reprogramming erases leukaemia-specific methylation pattern To understand the role of DNA methylation during CML development, we generated Leukaemia-iPS (LiPS) cells from two CML cell lines, K562 and KBM7, as well as from human CML primary bone marrow cells obtained from a BCR-ABL-positive CML patient. Leukaemia cells were transduced as previously reported [13] , [20] . Two weeks after infection, colonies with typical human ES-like morphology were picked and expanded on mouse embryonic fibroblast feeder layers resulting in stable ES-like cell lines: LiPS1-K562 and LiPS2-K562, both derived from the K562 cell line, and CML-LiPS1 and CML-LiPS2, derived from primary CML cells. In addition, we included the previously characterized KBM7 cell line and its reprogrammed counterpart in our analysis [15] . Remarkably, reprogrammed primary CML cells still preserved the BCR-ABL oncogene ( Supplementary Fig. 1c and [15] ). A comprehensive SNP array analysis confirmed that LiPS clones derived from K562 and KBM7 cell lines retained the same genetic alterations as the parental leukaemia cells ( Supplementary Fig. 2 and Supplementary Data 1-2 ) ruling out the possibility that an essentially normal subclone or contaminating cell was selected during reprogramming. Having established several LiPS cell lines, we proceeded to test whether cellular reprogramming was sufficient to reset DNA methylation of the parental leukaemic cells. Genomic DNA methylation profiles of K562, KBM7, primary CML cells and of the respective LiPS clones were assessed by Reduced Representation Bisulfite Sequencing (RRBS), which has been shown to provide high sensitivity and specificity for detecting cancer-specific changes in DNA methylation not only in CpG islands but also throughout genes and in repetitive regions [21] , [22] . Compared with human ES cells, CD34 + -derived iPS cells (CD34 + -iPS) and CD34 + cells, K562 and KBM7 cell lines exhibited widespread hypermethylation throughout the genome, including CpG islands, genes and promoters ( Fig. 1a ) as well as across families of repetitive elements. Primary CML cells also demonstrated significant hypermethylation in CpG islands, gene, and promoter regions, although to a lesser extent than in the cell lines. Compared with pluripotent cells, primary CML cells demonstrated hypermethylation across families of repetitive elements, similarly to CD34 + cells ( Fig. 1a ). 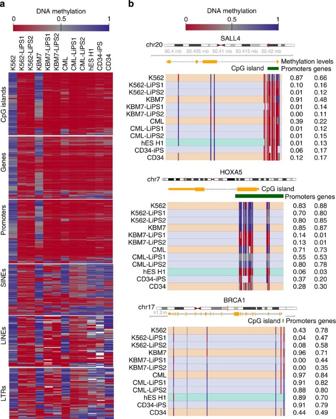Figure 1: Reprogramming erases the aberrant DNA methylation patterns in LiPS cells. (a) DNA methylation profile of K562 and KBM7 cell lines, primary patient-derived CML cells, their corresponding LiPS clones, as well as human ES cells, CD34+-iPS and primary CD34+cells from healthy donors. Each column of the heat map represents the average over two biological replicates. The heat map visualizes DNA methylation levels, with red colour indicating low levels of DNA methylation and blue colour indicating high levels. White colour indicates DNA regions not covered by RRBS analysis. For each genomic region type, shown are the 2% of regions that scored highest according to a ranking score in differential analysis comparing the group of K562, KBM7 and primary CML samples to the group including all derived iPS cell lines (see also the Methods section). (b) DNA methylation profile of theSALL4gene locus, hypermethylated in all the leukaemia cells and demethylated after reprogramming (upper panel). DNA methylation profiles ofHOXA5andBRCA1gene loci are shown in the middle and lower panels, respectively. Each row represents a sample, while each column represents a CpG dinucleotide. Blue colour indicates high DNA methylation levels and red colour indicates low methylation levels. CpG islands are annotated with green bars. Mean promoter and gene methylation levels are indicated on the right. Figure 1: Reprogramming erases the aberrant DNA methylation patterns in LiPS cells. ( a ) DNA methylation profile of K562 and KBM7 cell lines, primary patient-derived CML cells, their corresponding LiPS clones, as well as human ES cells, CD34 + -iPS and primary CD34 + cells from healthy donors. Each column of the heat map represents the average over two biological replicates. The heat map visualizes DNA methylation levels, with red colour indicating low levels of DNA methylation and blue colour indicating high levels. White colour indicates DNA regions not covered by RRBS analysis. For each genomic region type, shown are the 2% of regions that scored highest according to a ranking score in differential analysis comparing the group of K562, KBM7 and primary CML samples to the group including all derived iPS cell lines (see also the Methods section). ( b ) DNA methylation profile of the SALL4 gene locus, hypermethylated in all the leukaemia cells and demethylated after reprogramming (upper panel). DNA methylation profiles of HOXA5 and BRCA1 gene loci are shown in the middle and lower panels, respectively. Each row represents a sample, while each column represents a CpG dinucleotide. Blue colour indicates high DNA methylation levels and red colour indicates low methylation levels. CpG islands are annotated with green bars. Mean promoter and gene methylation levels are indicated on the right. Full size image DNA methylation levels were substantially decreased throughout the genome in the LiPS cells as compared with their parental leukaemic cell types, demonstrating the ability of cellular reprogramming to reset aberrant methylome ( Fig. 1a ). Overall, the LiPS clones acquired DNA methylation patterns that were similar but not identical to those of ES cell lines and CD34+iPS, supporting the notion of cell-of-origin-specific ‘epigenetic memory’ in many types of induced pluripotent cells [23] , [24] . Indeed, through genome-scale DNA methylation analysis, we identified LiPS-specific DNA methylation changes of relevant pluripotent and hematopoietic-associated genes. Pluripotent genes such as SALL4 were reactivated in LiPS and exhibited decreased DNA methylation levels, particularly at the promoter regions consistent with the well-established role of DNA demethylation as a key event in cellular reprogramming ( Fig. 1b and Supplementary Fig. 3 ) [18] . Epigenetic reprogramming affected not only pluripotency-associated genes but also other genomic loci, that is, hematopoietic transcription factors or tumour suppressor genes highly methylated across leukaemia cells and responding to cellular reprogramming with different extent of LiPS demethylation ( Fig. 1b ). Characterization of differentially methylated regions in CML To characterize the changes in DNA methylation that are induced by the reprogramming of CML cells to pluripotency, we used the RRBS data to bioinformatically identify differentially methylated regions (DMRs) between LiPS clones and the cells they were derived from (see Materials and Methods). Among the 500 strongest DMRs that are associated with gene promoters, the vast majority were hypermethylated in CML cells as compared with the derived LiPS cells ( Fig. 2a ). This observation is consistent with the increased levels of promoter methylation that are common among cancer cells. To better understand the biological functions of the genes that are characterized by differential promoter methylation, we performed gene ontology enrichment analyses. The 500 gene promoters hypermethylated in CML cells as compared with LiPS cells were significantly enriched for functional categories associated with development, differentiation and signalling ( Fig. 2b and Supplementary Table 1 ), suggesting that certain aspects of these stem cell-associated processes may be silenced by DNA methylation in CML cells. In contrast, the 500 gene promoters strongly hypermethylated in LiPS as compared with CML cells were enriched for hematopoietic regulatory gene categories such as lymphocyte activation and immune response ( Fig. 2c and Supplementary Table 1 ), the latter recently shown to be attenuated in iPS cells [25] , [26] . 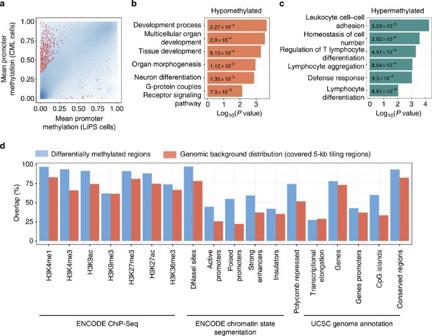Figure 2: Characterization of DMRs distinguishing CML cells from their reprogrammed counterparts. (a) Scatterplot comparing mean promoter methylation in CML cells with their derived LiPS cell lines. The blue colour gradient depicts point density. The 500 promoters with highest combined ranking of absolute/relative differential methylation and statistical significance are depicted in red. (b–c)Pvalues for significant Gene Ontology terms enriched among the 500 most highly ranking hypomethylated (red) and hypermethylated (green) gene promoters in reprogrammed cells relative to CML cells. (d) Overlap with genomic and epigenomic features in an EpiExplorer analysis27. The 500 most highly ranking differentially methylated tiling regions (blue) are compared with a background of 72,469 of 5-kb tiling regions covered by RRBS (red). The ChIP-seq peak tracks are from the ENCODE project for the GM12878, HMEC, NHLF, NHEK, HUVEC and H1 ES cell lines, chromatin state segmentations are based on chromHMM47and the gene, gene promoter (TSS−5 kb to TSS+1 kb), CpG islands, repeat and conserved locus annotation are from the UCSC Genome Browser. Overlaps of at least 1 bp are shown as percentage of all regions. Figure 2: Characterization of DMRs distinguishing CML cells from their reprogrammed counterparts. ( a ) Scatterplot comparing mean promoter methylation in CML cells with their derived LiPS cell lines. The blue colour gradient depicts point density. The 500 promoters with highest combined ranking of absolute/relative differential methylation and statistical significance are depicted in red. ( b – c ) P values for significant Gene Ontology terms enriched among the 500 most highly ranking hypomethylated (red) and hypermethylated (green) gene promoters in reprogrammed cells relative to CML cells. ( d ) Overlap with genomic and epigenomic features in an EpiExplorer analysis [27] . The 500 most highly ranking differentially methylated tiling regions (blue) are compared with a background of 72,469 of 5-kb tiling regions covered by RRBS (red). The ChIP-seq peak tracks are from the ENCODE project for the GM12878, HMEC, NHLF, NHEK, HUVEC and H1 ES cell lines, chromatin state segmentations are based on chromHMM [47] and the gene, gene promoter (TSS−5 kb to TSS+1 kb), CpG islands, repeat and conserved locus annotation are from the UCSC Genome Browser. Overlaps of at least 1 bp are shown as percentage of all regions. Full size image Beyond this gene promoter centric analysis of the potential biological functions of differential DNA methylation between CML cells and LiPS cells, we also investigated the co-localization of DNA methylation changes with other epigenetic and regulatory mechanisms throughout the genome. To that end, we repeated the differential DNA methylation analysis on the 5-kb tiling regions spanning the whole genome, and we used the EpiExplorer software [27] to compare the 500 most DMRs with the background of all tiling regions. This analysis revealed that DMRs are enriched for epigenetic marks associated with gene regulatory sequences including promoters and enhancers. Further, consistent with previous studies demonstrating a strong association between Polycomb binding in pluripotent cells and hypermethylation in cancer [28] , [29] , we observed that the CML hypermethylated regions were highly enriched for Polycomb binding sites ( Fig. 2d ). Overall, these observations confirm that CML reprogrammed into LiPS cells undergo epigenome reprogramming that erases characteristic patterns of cancer-associated DNA methylation while establishing characteristic DNA methylation patterns of pluripotent cells. Reprogramming restores myeloid differentiation of CML cells To assess whether epigenetic reprogramming observed in LiPS cells coincides with phenotypic changes in their oncogenic potential, we applied in vitro and in vivo strategies using both primary human CML cells and the CML model cell line K562, chosen for its high efficiency of engraftment in xenotransplantation approaches. By co-culture with OP9 stroma cells [30] ( Supplementary Fig. 4a ), we demonstrated that CML-LiPS-derived CD45 + /CD34 + cells reacquire myeloid and erytroid differentiation capabilities giving rise to CD15 + /CD14 + /GlyA + cells, despite the presence of BCR-ABL oncogene ( Supplementary Fig. 4a-d ). With a similar OP9 co-culture we proved that K562-LiPS-derived CD45 + cells exhibit a well-differentiated monocyte/macrophage phenotype in contrast with the leukaemia counterpart, locked into an undifferentiated cellular state ( Fig. 3a and Supplementary Fig. 4e ). Indeed, while the parental leukaemia and LiPS cells showed low expression of the hematopoietic transcription factor CEBPA , the purified CD45 + LiPS-derived cells demonstrated the reactivation of this critical differentiation-associated gene locus and increase of its levels of expression ( Supplementary Fig. 4f-g ). Remarkably, when K562-LiPS-derived CD45 + cells and the parental leukaemia cells (20,000 per mouse) were injected into immunocompromised NOD.Cg-Prkdc scid Il2 rgtm1Wjl /SzJ (NSG) mice, all mice (=3) transplanted with leukaemic cells developed the disease and died within 30 days after the injection. In contrast, seven out of the eight mice transplanted with LiPS-derived CD45 + cells, regardless the successful engraftment, did not show any sign associated with a leukaemic phenotype, that is, spleen infiltration as observed in case of K562, during the entire 80 days of monitoring period ( Fig. 3b,c ). 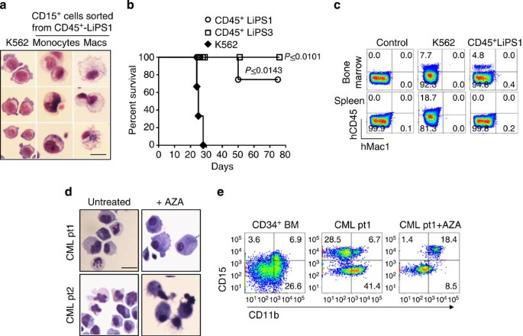Figure 3: Reprogramming restores myeloid differentiation decreasing the malignancy of leukaemia cells. (a) CD45+CD15+cells derived from LiPS 1 clone revealing a typical morphology of terminally differentiated monocytes (centre) and macrophages (right; scale bars, 20 μm). (b) Survival curve of NSG mice transplanted with K562 cells (n=3), LiPS1-derived CD45+cells (n=4) and CD45+ LiPS3 cells (n=4;*P<0.05; **P<0.01 and ***P<0.001; Mantel–Cox survival test). (c) FACS analysis showing engraftment of K562 cells, LiPS-derived CD45+cells and a negative control in NSG mice. Indicated are the percentages of CD45+cells. (d) Primary cells from two CML patients acquiring typical morphology of terminally differentiated monocytes after AZA treatment. (e) FACS analysis showing the high expression of myeloid differentiation marker CD11b and CD14 in primary CML cells after AZA treatment. Figure 3: Reprogramming restores myeloid differentiation decreasing the malignancy of leukaemia cells. ( a ) CD45 + CD15 + cells derived from LiPS 1 clone revealing a typical morphology of terminally differentiated monocytes (centre) and macrophages (right; scale bars, 20 μm). ( b ) Survival curve of NSG mice transplanted with K562 cells ( n =3), LiPS1-derived CD45 + cells ( n =4) and CD45+ LiPS3 cells ( n =4; *P <0.05; ** P <0.01 and *** P <0.001; Mantel–Cox survival test). ( c ) FACS analysis showing engraftment of K562 cells, LiPS-derived CD45 + cells and a negative control in NSG mice. Indicated are the percentages of CD45 + cells. ( d ) Primary cells from two CML patients acquiring typical morphology of terminally differentiated monocytes after AZA treatment. ( e ) FACS analysis showing the high expression of myeloid differentiation marker CD11b and CD14 in primary CML cells after AZA treatment. Full size image Finally, to investigate the potential contribution of DNA methylation in CML pathogenesis, we applied 5-Azacytidine (AZA) treatment to primary CML cells. On treatment with AZA, we observed a skew in differentiation towards the granulocyte and monocyte/macrophage lineages, as shown by the presence of CD15 + and CD11b + cells, as compared with the untreated cells ( Fig. 3d,e ), suggesting that DNA methylation abnormalities cooperate in disrupting hematopoietic differentiation during CML development and progression. BCR-ABL induction reprograms DNA methylation pattern Our observations prompted us to investigate the functional relationship between the presence or absence of BCR-ABL oncogene and DNA methylation response. To address this question, we took advantage of a transgenic murine model in which BCR-ABL expression can be conditionally induced and reversibly repressed [19] . Indeed previous studies, both in cell culture and in vivo , have shown that the overexpression of specific oncogenes such as MLL-AF9 and mutant IDH1 are capable of inducing epigenetic reprogramming comparable to that observed in human disease [31] , [32] , [33] . In our model, BCR-ABL is under the control of the 3′ enhancer of the murine SCL (stem cell leukaemia) gene, thus allowing BCR-ABL expression mainly in the hematopoietic stem sell (HSC) compartment and leading to development of a chronic myeloproliferative disorder similar to human CML [19] . Induction of BCR-ABL expression by the withdrawal of tetracycline from the drinking water leads to a significant increase in Gr1 and Mac1 positive myeloid population (leukaemic mice). This phenotype can be reversed when tetracycline is added to the water (rescued mice), thus confirming a direct correlation between BCR-ABL presence and the expansion of that population ( Fig. 4a and ref. 19 ).Using this mouse model, we analysed DNA methylation patterns in the HSCs population harvested from three distinct groups of mice: (i) the non-induced BCR-ABL mice (control); ii) the induced BCR-ABL mice (leukaemic) and (iii) the repressed BCR-ABL mice (rescued). Leukaemic mice showed moderate increase of CpG islands DNA methylation levels, indicating that a single oncogenic fusion protein can trigger characteristic perturbations of DNA methylation in a highly defined mouse model ( Fig. 4b ). Upon BCR-ABL activation, the leukaemic mice acquired aberrant DNA methylation at several gene loci, one example being the hematopoietic transcription factor Hoxb1 ( Fig. 4c,d and Supplementary Table 2 ). Remarkably, the repression of BCR-ABL led to the widespread reversion of the BCR-ABL-induced changes in DNA methylation, supporting the hypothesis that BCR-ABL triggers DNA methylation changes. This observation could be explained by transcription factors and epigenetic regulator proteins directly downstream of BCR-ABL influencing DNA methylation, but it could also be a reflection of a broader change in epigenetic cell states when BCR-ABL transforms cells. 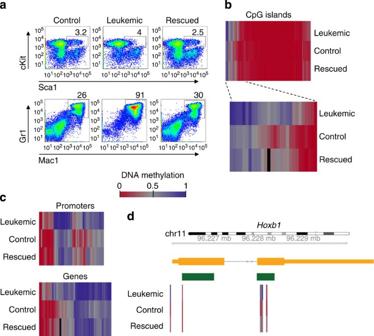Figure 4: BCR-ABL activation induces the aberrant DNA methylation pattern in murine HSCs. (a) FACS analysis of BCR-ABL transgenic murine bone marrow mononuclear cells in which the BCR-ABL oncogene is not expressed (‘control’), is expressed (‘leukaemic’) or repressed after previous expression (‘rescued’). Leukaemic mice showed moderate expansion of the HSCs population cKit+Sca1+and a strong expansion of the Mac1+Gr1+myeloid population compared with control and rescued animals. (b) DNA methylation analysis of CpG islands in the Lin−cKit+Sca1+population of BCR-ABL transgenic mice with different status of oncogene expression. Zoomed-in region shows example of CpG islands differentially methylated between leukaemic, control and rescue mice. Each row represents the average of two biological replicates. Each column represents a complete CpG island. Blue: high methylation, red: low methylation. White colour indicates DNA regions not covered by RRBS analysis. (c) Heat map visualizing genes and promoters hypermethylated in leukaemic mice versus control and rescued ones. (d) High-resolution view of DNA methylation of theHoxb1gene locus, which was hypermethylated in leukaemic mice as compared with the control mice. Each row represents the average of two biological replicates; each column represents a single CpG dinucleotide. Figure 4: BCR-ABL activation induces the aberrant DNA methylation pattern in murine HSCs. ( a ) FACS analysis of BCR-ABL transgenic murine bone marrow mononuclear cells in which the BCR-ABL oncogene is not expressed (‘control’), is expressed (‘leukaemic’) or repressed after previous expression (‘rescued’). Leukaemic mice showed moderate expansion of the HSCs population cKit + Sca1 + and a strong expansion of the Mac1 + Gr1 + myeloid population compared with control and rescued animals. ( b ) DNA methylation analysis of CpG islands in the Lin − cKit + Sca1 + population of BCR-ABL transgenic mice with different status of oncogene expression. Zoomed-in region shows example of CpG islands differentially methylated between leukaemic, control and rescue mice. Each row represents the average of two biological replicates. Each column represents a complete CpG island. Blue: high methylation, red: low methylation. White colour indicates DNA regions not covered by RRBS analysis. ( c ) Heat map visualizing genes and promoters hypermethylated in leukaemic mice versus control and rescued ones. ( d ) High-resolution view of DNA methylation of the Hoxb1 gene locus, which was hypermethylated in leukaemic mice as compared with the control mice. Each row represents the average of two biological replicates; each column represents a single CpG dinucleotide. Full size image In summary, these data demonstrate the functional effect of a single genetic lesion in determining the aberrant methylome state, suggesting that epigenetic alterations act as a secondary precipitating event during leukaemia development. 5-Azacytidine reduces BCR-ABL cells oncogenic potential To test whether the inhibition of BCR-ABL-induced aberrant DNA methylation could restore normal hematopoiesis during leukaemogenesis, six leukaemic mice per group were treated for 4 weeks with AZA (2 mg kg −1 ) or with the tyrosine kinase inhibitor imatinib (200 mg kg −1 ; IM, first line treatment for CML), respectively. Mice treated with AZA exhibited no expansion of the Mac1 + Gr1 + myeloid population as compared with the untreated counterpart, closely mimicking the results observed for the IM-treated group used as a positive control. Furthermore, both AZA- and IM-treated mice displayed normal lymphopoiesis, absent in the untreated controls ( Supplementary Fig. 5a ). These data indicate that despite their different mechanisms of action, both AZA, at the epigenetic level by correcting aberrant DNA methylation and IM at the genetic level by blocking the BCR-ABL oncogene, are capable of re-establishing normal hematopoiesis. To further evaluate the contribution of aberrant DNA methylation to leukaemia development in vivo , 44 irradiated B6.SJL- Ptprc a Pepc b /BoyJ (pep boys) congenic recipient mice were transplanted with murine BCR-ABL leukaemic bone marrow cells. Eight to ten mice were randomly assigned to five groups: control (not leukaemic); leukaemic untreated, treated with AZA (2 mg kg −1 ); or IM (200 mg kg −1 ) or combination of the two drugs IM and AZA. The treatment was administered for 4 weeks ( Supplementary Fig. 5b ) and the mice were followed up for a period of up to 150 days. The untreated mice developed leukaemia (as expected) with a median survival of 41 days. Strikingly, the AZA treatment provided longer survival (median survival 100 days; P =0.0008) than the IM treatment (median survival: 56 days; P =0.03) as compared with the untreated mice. Unfortunately, the combination of AZA and IM, at their standard dosages, resulted in haematological and gastrointestinal toxicity for the mice that did not allow us to make any conclusive observation on the potential benefits of using combination of the drugs to correct the leukaemic phenotype. Future studies will be necessary to assess optimal dosage range and scheduling mode to: (1) reduce the toxicity and (2) understand the potential synergic effect of the two drugs ( Fig. 5b ). Moreover, the AZA treatment efficiently targeted the stem cell compartment (LSK population from the CD45.2+ donor cells), restoring expression and promoting demethylation of loci differentially methylated between control and sick mice ( Supplementary Data 2 ), such as the Gdf3 (Growth differentiation factor 3) ( Supplementary Fig. 6 ), a promising target of the BCR-ABL oncogene. 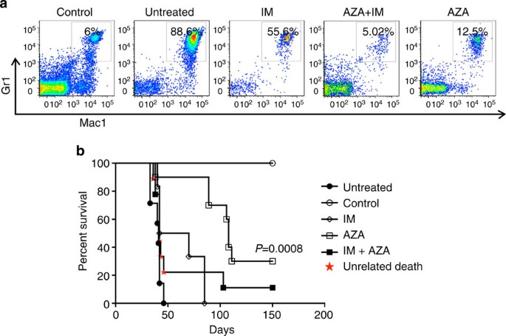Figure 5: 5-Azacytidine reduces the oncogenic potential of BCR-ABL-expressing cells. (a) Peripheral blood FACS analysis of BCR-ABL transgenic mice expressing BCR-ABL shows strong reduction of the Mac1+and Gr1+myeloid population in mice treated with imatinib, AZA or combination of the two drugs. (b) Survival curve of B6.SJL-PtprcaPepcb/BoyJ (pep boys) congenic recipient mice transplanted with BCR-ABL leukaemic bone marrow shows prolonged survival rate upon AZA treatment as compared with imatinib group and untreated mice. Between 8–10 mice (diagram of treatment shown inSupplementary Fig. 5b) were used per each group. (*P<0.05; **P<0.01 and ***P<0.001; Mantel-Cox Survival Test). Figure 5: 5-Azacytidine reduces the oncogenic potential of BCR-ABL-expressing cells. ( a ) Peripheral blood FACS analysis of BCR-ABL transgenic mice expressing BCR-ABL shows strong reduction of the Mac1 + and Gr1 + myeloid population in mice treated with imatinib, AZA or combination of the two drugs. ( b ) Survival curve of B6.SJL- Ptprc a Pepc b /BoyJ (pep boys) congenic recipient mice transplanted with BCR-ABL leukaemic bone marrow shows prolonged survival rate upon AZA treatment as compared with imatinib group and untreated mice. Between 8–10 mice (diagram of treatment shown in Supplementary Fig. 5b ) were used per each group. (* P <0.05; ** P <0.01 and *** P <0.001; Mantel-Cox Survival Test). Full size image Taken together, these data indicate that DNA methylation aberrations play a critical role in CML development, supporting the relevance of DNA methylation modulating drugs as therapeutic options. This study analysed the interconnection and functional relevance of genetic and epigenetic alterations in CML. By deriving genetically matched but epigenetically distinct LiPS cell lines from CML cell lines and human primary CML cells, and by using an inducible mouse model of CML, we show that: (1) genetic and epigenetic alterations are both required to maintain the leukaemic potential, and (2) that the BCR-ABL fusion protein is able to trigger DNA methylation changes that can act as a secondary event and contribute to leukaemia formation. Using nuclear reprogramming as an ‘epigenetic tool’ we were able to erase aberrant DNA methylation from leukaemia cells, thereby delaying the onset of the malignancy. Among the leukaemia-specific DMRs, less than half were associated with promoters, whereas the vast majority corresponded to specific histone marks such as enhancer-associated H3K4me1 and promoter-associated H3K4me3. Interestingly, genes hypermethylated in LiPS compared with CML cells belonged to functional categories of lymphocyte activation and immune response. It has been shown that iPS cells are defective in their antiviral response as a result of the downregulation of key genes involved in immune response [25] , [26] . Similarly, attenuated antiviral response reported in human ES cells is restored by differentiation, suggesting that the impaired antiviral response of iPS cells likely stemmed from the pluripotent state and might promote cell pluripotency [25] , [26] , [34] . Our data show that the mice transplanted with CD45 + cells derived from LiPS do not develop leukaemia within the 80 days monitoring time ( Fig. 3b ). In particular, we demonstrated that leukaemia progression was susceptible not only to the genetic inhibition of the driving oncogene but also to the inhibition of the secondary DNA methylation changes, which provides strong evidence for the cooperative role of both genetic and epigenetic alterations in leukaemia. In a related study focusing on glioblastoma, Stricker et al . [35] recently demonstrated that the reprogramming of glioblastoma cells was also able to erase aberrant DNA methylation. But in contrast to our observations for CML, these induced epigenetic changes were insufficient to compromise oncogenic potential, and neural progenitors derived from the reprogrammed glioblastoma remained highly malignant. This important difference between glioblastoma and CML supports the relevance of aberrant DNA methylation specifically in CML, consistent with the much lower rates of genetic alterations in leukaemia compared with glioblastoma [36] and with the history of successful use of DNA methylation inhibitors in leukaemias. This conclusion is further supported by comparing our results in CML with a recent study focusing on cells derived from Ewing sarcoma patients, which is a solid tumour driven by an oncogenic fusion protein EWS-FLI1. On knockdown, Tomazou et al . [37] observed widespread changes in histone acetylation and histone methylation, whereas DNA methylation patterns were largely unaffected. Consistent with this observation, AZA had a much weaker effect in EWS-FLI1-expressing cells than histone deacetylase inhibitors, whereas the functional impact of AZA on BCR-ABL-expressing cells in our mouse model was striking and even exceeded those observed for imatinib. Overall, these results highlight the specific relevance of aberrant DNA methylation in CML, which are driven by BCR-ABL expression and are at the same time essential for maintaining a strong leukaemic phenotype in a mouse model. This study provides a rationale for broadly exploring the use of demethylating agents as adjuvant treatments in leukaemia, even in subtypes with recurrent and well-characterized genetic abnormalities such as BCR-ABL. Cell cultures and LiPS cells generation Human K562 leukaemia cells (ATCC CCL-243) and U937 cells (ATCC CRL-1593.2) were cultured following the manufacturer’s instructions. KBM7 cells were a kind gift from the T. R. Brummelkamp laboratory. They were cultured in DMEM 10% fetal bovine serum (FBS). iPS derived from CD34 + cells were a gift from the George Daley laboratory and were maintained in human ES cell media (Invitrogen) in the presence of FGF (Peprotech) and 20% of Replacement Serum (Invitrogen) as described in ref. 38 . Primary CML total bone marrow mononuclear cells were obtained after a written informed consent in accordance with the Declaration of Helsinki in agreement with the approved protocol from the review board of the S.Orsola-Malpighi Hospital, Bologna, Italy. Primary samples were cultured in QBSF-60 (Quality Biological), 20% FBS, SCF 50 μg ml −1 , TPO 20 μg ml −1 , Flt3 10 μg ml −1 , IL3 10 μg ml −1 . Retroviral infections were performed as described in refs 13 , 20 . In brief, cells were transduced with a pool of the four factors Oct4, Sox2, Klf4 and c-Myc in a ratio of 1:1:1:1 for a 72 h period. At day 4 post transduction, regular medium was switched to human ES cell media (Invitrogen) in the presence of FGF (Peprotech) and 20% of Replacement Serum (Invitrogen). After 15-16 days, human iPS-like colonies were morphologically identified, picked and mechanically disaggregated on irradiated mouse embryonic fibroblasts (Globalstem). CML primary cells were treated with 1 μM of 5-Azacytidine for 72 h to allow monocytic differentiation. In vitro differentiation Embryoid body (EB) formation was induced by culturing human LiPS in clumps in the absence of FGF in bacterial plates to avoid attachment to the bottom of the plates. To allow spontaneous endoderm formation, after 3–4 days, embryoid bodies were transferred onto 0.2% gelatin-coated glass six-well plates and cultured in differentiation medium (DMEM supplemented with 20% FBS, 2 mM l-glutamine, 0.1 mM 2-mercaptoethanol, nonessential amino acids and penicillin–streptomycin, all from Invitrogen) for 2 to 3 weeks. The medium was changed every other day. For mesoderm/cardiomyocyte differentiation, LiPS cells were maintained on gelatin-coated plates in differentiated medium supplemented with 100 μM ascorbic acid (Sigma). For ectoderm differentiation, EBs were cultured on laminin (Stemgent) coated six-well plates. In brief, after 4 days in EB medium as a floating culture, the cells were plated on laminin (Stemgent)-coated plates in N2B27 medium (Invitrogen), Sonic Hedgehog (0.1 μg μl −1 ) and FGF8 (100 ng ml −1 ; both from Peprotech), and maintained for 3 to 5 weeks in the absence of FGF2. The medium was changed every other day. Immunofluorescence analysis Cells were grown in six-well plates and fixed with 4% paraformaldehyde. The following antibodies were used: OCT4 (1:200; Abcam 19857), NANOG (1:200; Abcam 21624), Tra1-81 (1:200; Abcam 16289), Tra1-60 (1:200; Abcam 16288), Smooth Muscle Actinin (SMA; 1:200; Abcam 5694), Tuj1 (1:200; Covance MMS-435P) and α-fetoprotein (1:200; Dako A 0008). Secondary antibodies used were from Jackson Immunoresearch: DyLight 549-coniugated AffiniPure Goat Anti-Rabbit IgG (1:250; 111-505-303); DyLight 488-coniugated AffiniPure Donkey Anti-mouse IgG (1:250; 715-485-150) and were used according to the manufacturer’s guidelines. Images were taken using an Axiovert 200M microscope (Zeiss). Teratoma formation and analysis Between 2 and 10 million iPS cells were mechanically scraped, pelleted, resuspended in 100 μl of hES media and injected subcutaneously and intramuscularly into NOD.Cg- Prkdc scid Il2rg tm1Wjl /SzJ (NSG). Teratomas were harvested after 9 weeks, fixed overnight with 10% formaldehyde, embedded in paraffin, sectioned, HE stained and analysed using a BX40 microscope (Olympus). All the animal work and protocols were approved by the Institutional Animal Care and Use Committee of Beth Israel Deaconess Medical Center (Protocol #006-2014) and were performed in accordance with the guidelines set forth in the Guide for the Care and Use of Laboratory Animals of the National Research Council of the National Institutes of Health. Western blot analysis Cells (200,000–500,000) were washed twice in PBS and then lysed in 50 mM Tris/HCl buffer, pH 8.0, containing 150 mM NaCl, 1% Nonidet P-40, 2 μg ml −1 aprotinin, 1 μg ml −1 pepstatin, 2 μg ml −1 leupeptin and 1 mM Na 3 VO 4 . Equal amounts of extracted proteins (50 μg) were loaded and separated on SDS–PAGE (Invitrogen), and then transferred onto a nitrocellulose membrane (Schleicher & Schuell Biosciences, Sandford, ME). Immunodetection was performed using the following primary antibodies: anti-ABL (1:500; Millipore MABT203) and β-actin (1:2,000; Santa Cruz47778). Full western blot is presented as Supplementary Fig. 7a . Methylcellulose colony assay Methylcellulose colony formation assays were performed with Methocult H4434 (Stem Cell Technologies) according to the manufacturer’s instructions. CD34 + /CD45 + cells sorted from Bone Marrow or from in vitro differentiated CML-LiPS were suspended in a culture medium containing methylcellulose and plated onto 35-mm culture dishes at a density of 10 3 (BM-derived) or 10 4 (CML-LiPS derived) cells/dish, in triplicates. Colonies were counted after 2 weeks and processed for differentiation markers by fluorescence-activated cell sorting (FACS) after 3 weeks. SNP analysis The analysis was performed using Affymetrix 6.0 SNP arrays platform and then computationally using the Partek Genomics Suite. In brief, normalization using global median was first performed for array intensities cross all chips. Copy numbers and allele ratios were then estimated by comparison with a common reference to identify the copy number variations in the parental cell lines as well as the additional variations in copy numbers caused by reprogramming. Genomic segmentation was performed to smooth the data with the following parameters: 10 as the minimum of data points (SNPs), 0.001 as the cutoff for P value, 0.2 as the noise-to-signal cutoff. Reduced representation bisulfite sequencing RRBS was performed as it follows. Genomic DNA was isolated from K562, K562-LiPS1, K562-LiPS2, KBM7, KBM7-LiPS1, KBM7-LiPS2, primary CML, CML-LiPS1 and CML-LiPS2, CD34 + iPS and digested with MspI (NEB), a methylation-insensitive enzyme that cuts C’CGG sites independent of the DNA methylation status of the centre CpG. Digested DNA was size selected on a 4% NuSieve 3:1 Agarose gel (Lonza). For each sample, two slices containing DNA fragments of 40–120 bp and 120–220 bp, respectively, were excised from the unstained preparative portion of the gel. These two size fractions were kept apart throughout the procedure including the final sequencing. Pre-annealed Illumina adaptors containing 5’-methyl-cytosine instead of cytosine were ligated to ends of size-selected MspI fragments. Adapter-ligated fragments were bisulfite-treated using the Epitect kit (Qiagen). The products were PCR amplified, size selected and sequenced on the Illumina GA IIx at a reading length of 36 bp. Sequencing reads were mapped to the human genome assembly NCBI37/hg19 and mm9 for human and mouse data, respectively, using RRBSMAP [39] allowing two mismatches. Methylation levels were called using the BisSNP software [40] . RRBS data for human H1 ES line passage 37 and 38 and CD34 + cells were obtained from the Roadmap Epigenomics Project. Further processing was done using RnBeads ( http://rnbeads.mpi-inf.mpg.de/ ) [41] .In this analysis, promoter methylation was defined as the mean across all scores for CpGs within a window of −1,500 bp to +500 bp of the TSS of Ensembl-annotated genes. Differentially methylated sites were identified using a ranking-based approach taking into account statistical testing as well as absolute and relative differences in methylation levels between the two groups of samples. In brief, we defined a combined ranking score for a single CpG as the maximum, that is, worst, rank among the following three criteria: (a) absolute difference in group mean methylation levels, (b) absolute log ratios in group mean methylation levels and (c) P values originating from hierarchical linear models [42] . For genomic regions, such as CpG islands, genes, promoters, and so on, the combined ranking score was defined analogously based on (a) mean differences in mean methylation levels across all CpGs in a particular region (b) mean ratios of mean methylation levels across CpGs (c) combining the CpG specific P values using an extension of Fisher's method [43] . Full RnBeads analysis reports, including tables characterizing differential methylation, can be accessed at http://reprogramming-leukemia.computational-epigenetics.org/ . Bisulfite sequencing Methylation profiling of CEBPA , gene loci was performed using 1 μg of genomic DNA. For the analysis DNA was bisulfite converted using the EpiTect kit (Qiagen). The primers and PCR conditions for bisulfite sequencing are: F- OCT4 : 5′- TAG TTG GGA TGT GTA GAG TTT GAGA -3′, R- OCT4 : 5′- TAA ACC AAA ACA ATC CTT CTA CTC C -3′; F- CEBPA : 5′- TAG TTT YGT TAG TTT GGG GGG TTT -3′, R- CEBPA : 5′- TCT AAT CTC CAA ACT ACC CCT ATA -3′; F- CEBPA coding region: 5′- AGG TTA AGG YGG TTG TGG GTT TTA -3′; R- CEBPA : 5′- CCA ACT ACT TAA CTT CAT CCT CCT -3′. PCR products were gel purified (Qiagen) and cloned into a plasmid vector, pGEM-T Easy Vector System (Promega). Sequencing results were analysed using BiQ Analyzer software [44] . Methylation-specific PCR Genomic DNA from ∼ 4−10 × 10 3 CD45 + /Lineage − / cKit + / Sca1 + cells was directly bisulfite converted using the EZ DNA Methylation kit (Zymo Research) according to the manufacturer's instructions. Bisulfite-treated genomic DNA was amplified using AmpliTaq Gold 360 Master Mix (Life Technology) and methylated (M) or unmethylated (UM)-specific primer sets, designed with the MethPrimer software [45] . Gdf3-M Forward: 5′- TTA TAG GTT TTA ATT TGT GTT TCG C -3′; Gdf3-M Reverse: 5′- AAT TTT TCT CTA ATA AAC CCT CGA A -3′; Gdf3-UM Forward: 5′- ATA GGT TTT AAT TTG TGT TTT GTG T -3′ and Gdf3-UM Reverse 5′- AAT TTT TCT CTA ATA AAC CCT CAA A -3′. Integral gel presented in Supplementary Fig. 7b . In vitro hematopoietic differentiation Embryoid bodies were produced by scraping of confluent LiPS cells and cultured in suspension in EB medium (90% DMEM, 10% FBS) for 96 h. Embryoid bodies were then placed over a feeder layer of confluent OP9 stromal cells and allowed to attach. The medium used for the first 48 h of differentiation was 50% EB medium and 50% hematopoietic differentiation medium. The hematopoietic differentiation medium was prepared with QBSF-60 serum-free medium (Quality Biological Inc) supplemented with cytokines BMP4 (10 ng ml −1 ), VEGF (10 ng ml −1 ), SCF (25 ng ml −1 ), FGF (10 ng ml −1 ), TPO (20 ng ml −1 ) and Flt ligand (10 ng ml −1 ; all from Peprotech). After 48 h, cells were cultured with hematopoietic differentiation medium, with medium changes every 48 h until the end of the differentiation protocol. At day 26, OP9 and embryoid bodies were collected by trypsinization (0.05% trypsin), washed and labelled for the cytofluorimetric analysis. FACS analysis and sorting Cells were suspended in Ca ++ Mg ++ -free PBS containing 2% (vol/vol) FBS (Globalstem). Human hematopoietic progenitors cells were identified by labelling with CD45-PE (1:50; clone HI30) and or CD34-APC (1:50; clone 561) while mature phenotypes were analysed using CD15-Pacific Blue (monocytes and granulocytes) (1:50; clone W6D3/HI98), CD14-FITC (monocytes and macrophages clone 1:50; M5E2); CD11b (1:50; ICRF44; macrophages) and Glycophorin-PECy5 (red blood cell membrane), and erythroid precursors (1:50; Clone HIR2; all from Biolegend). Murine hematopoietic cells were identified using the following antibodies: Mac1/CD11b-PECy7 (1:200; clone M1/70), Gr1-PE (1:200; clone 8C5), B220-PECy5 (1:100; clone RA3-6B2), Sca1-APC (1:100; clone E13-161-7), c-Kit-APCCy7 (1:100; clone 2B8): CD45.1-APC (1:100; clone A20) and CD45.2-FITC (1:100; clone 104; all from Biolegends). All antibodies were incubated at the concentration suggested by the manufacturer for 30 min on ice. Non-specific signals and dead cells were excluded by appropriate fluorochrome-conjugated isotype and propidium iodide staining, respectively. Cell fluorescence was analysed with the FACSAria II (Becton Dickinson). Quantitative reverse transcription PCR Total RNA was isolated from cells using TRIzol reagent (Invitrogen) and RNeasy Plus Mini Kit (Qiagen). Genomic DNA was eliminated with RNase-free DNase 1 (Roche), and total RNA was then subjected to another round of purification by phenol solution with pH4.3±0.2 (Sigma-Aldrich). For pluripotent gene expression analysis, cDNA was generated by SuperScript II reverse transcriptase (Invitrogen) with random hexamers (Invitrogen) from 1 μg of total RNA, and real-time PCR was performed with GoTaq qPCR Master Mix (Promega). Expression of CEBPA was quantified using Taqman one-step reverse transcription (RT)-PCR master mix (Applied Biosystems) relative to β-Actin. Primers used for CEBPA qRT-PCR were FW 5′- TCG GTG GAC AAG AAC AG -3′; REV 5′- GCA GGC GGT CAT TG -3′; Taqman Probe 5′- FAM ACA AGG CCA AGC AGC GC -3′. β-ACTIN was purchased from Applied Biosystem. Primers employed for BCR-ABL detection in qRT-PCR were: FW 5′- GCA TTC CGC TGA CCA TCA AT -3′; REV 5′– TGG GTC CAG CGA GAA GGT T -3′; probe 5′- FAM-CCA GTA GCA TCT GAC TTT GAG CCT CAG GG -TAMRA-3′ (ref. 46 ). For Gdf3 RNA was isolated from whole bone marrow mononuclear cells or CD45.2 + /LSK cells using TRIzol reagent (Invitrogen) and RNeasy mini kit (QIAGEN). cDNA was synthesized with Superscript First-Strand Synthesis System according to manufacturer's instructions (Invitrogen). qPCR was performed with SYBR reagent (Bio-Rad). Primers used were: Gdf3_F1 (Forward): 5′- GAA CCT GCT TCA GCT TCT CC -3′; Gdf3_R1 (Reverse): 5′- CCA TGG TCA ACT TTG CCT TT -3′. Gdf3 expression levels were normalized to that of Gapdh: Forward 5′- CCA GCC TCG TCC CGT AGA C -3′; Reverse 5′- CCC TTG ACT GTG CCG TTG -3′. Transplantation of immunocompromised and B6.SJL- Ptprc a Pepc b /BoyJ Sorted LiPS-derived CD45 + cells and K562 cells were transferred by intra-orbital injection into sublethally irradiated (150 cGy) 6-week-old recipient NSG mice (20,000 cells per mice). Transplanted mice were sacrificed for isolation of bone marrow and spleen. Transplantation was performed in quadruplicate for LiPS 1 clone and K562 and in triplicate for LiPS3 clone. 1 × 10 6 whole bone marrow cells obtained from SCL-tTA/BCR-ABL transgenic mice were transplanted by intra-orbital injection into 44-six-week-old CD45.1 B6.SJL-Ptprca Pepcb/BoyJ congenic mice lethally irradiated. Tetracycline was maintained in the drinking water for 3 weeks after transplantation. BCR-ABL expression was induced by the withdrawal of tetracycline and 2 weeks after BCR-ABL induction, treatment was started. Mice were randomly assigned to five groups: Control (Bcr-Abl un-induced); untreated (Bcr-Abl induced); IM (Bcr-Abl induced, treated with imatinib); AZA (Bcr-Abl induced, treated with 5-Azacytidine); IM+AZA (Bcr-Abl induced, treated with imatinib and 5-Azacytidine). The IM group received imatinib at the dosage of 200 mg kg −1 by gavauge, every other day. The AZA group received 5-Azacytidine by intraperitoneal injection at the dosage of 2 mg kg −1 every other day. The IM-AZA group received a combination of imatinib, 200 mg kg −1 by gavage, and 5-Azacytidine by intraperitoneal injection at the dosage of 2 mg kg −1 every other day. Mice were followed up for 150 days. Statistical analysis Survival curves were analysed using the Kaplan–Meier method. Differences in the survival curves were evaluated with the log-rank test. Values of P ≤0.05 were considered statistically significant. Statistical analyses of qRT-PCR were performed with paired two-tailed Student’s t -test. Error bars indicate mean ( n ⩾ 3)±standard deviation (s.d. ). Accession codes : RRBS data have been deposited in the gene expression omnibus (GEO) database under the accession number GSE50456 . How to cite this article: Amabile, G. et al . Dissecting the role of aberrant DNA methylation in human leukaemia. Nat. Commun. 6:7091 doi: 10.1038/ncomms8091 (2015).